The matricellular protein CCN1 mediates neutrophil efferocytosis in cutaneous wound healing Neutrophil infiltration constitutes the first step in wound healing, although their timely clearance by macrophage engulfment, or efferocytosis, is critical for efficient tissue repair. However, the specific mechanism for neutrophil clearance in wound healing remains undefined. Here we uncover a key role for CCN1 in neutrophil efferocytosis by acting as a bridging molecule that binds phosphatidylserine, the ‘eat-me’ signal on apoptotic cells and integrins α v β 3 /α v β 5 in macrophages to trigger efferocytosis. Both knockin mice expressing a mutant CCN1 that is unable to bind α v β 3 /α v β 5 and mice with Ccn1 knockdown are defective in neutrophil efferocytosis, resulting in exuberant neutrophil accumulation and delayed healing. Treatment of wounds with CCN1 accelerates neutrophil clearance in both Ccn1 knockin mice and diabetic Lepr db/db mice, which suffer from neutrophil persistence and impaired healing. These findings establish CCN1 as a critical opsonin in skin injury and suggest a therapeutic potential for CCN1 in certain types of non-healing wounds. Wound healing encompasses a highly coordinated series of events requiring the interaction of various cell types to achieve tissue integrity and homeostasis after injury. To this end, wound repair proceeds in three overlapping but functionally distinct phases—initiating with an inflammatory phase marked by infiltration of neutrophils and macrophages, followed by a proliferative phase that includes tissue formation and extracellular matrix deposition and concluding with a maturation phase that brings about matrix remodelling and resolution of the granulation tissue [1] , [2] . Inflammation begins immediately after wounding, when blood clotting with entrapped platelets and neutrophils release a host of factors that amplify the coagulation cascade and stimulate further recruitment of inflammatory cells. Neutrophils are the first immune cells to extravasate and infiltrate the wound, functioning to initiate debridement of devitalized tissues and to combat invading microbes by releasing reactive oxygen species, antimicrobial peptides, eicosanoids, proteases and neutrophil extracellular traps [3] , [4] . However, neutrophils must be eliminated in due course for wound healing to progress, as excessive or persistent neutrophil activity can cause further tissue damage and impede healing [5] , [6] . Indeed, chronic non-healing or slow-healing wounds, including diabetic wounds and pressure or venous ulcers, are often associated with prolonged inflammation and neutrophil persistence [7] , [8] , [9] . Unless their recruitment is sustained at the wound site, the short-lived, expended neutrophils undergo apoptosis and are largely removed by macrophages in situ within days [10] , [11] . Efferocytosis, or engulfment of apoptotic cells, stimulates macrophages to exhibit M2 phenotypes, which include the downregulation of pro-inflammatory cytokines and upregulation of anti-inflammatory and reparative cytokines such as transforming growth factor-β1 and interleukin-10 (ref. 12 ). Failure to eliminate apoptotic neutrophils often leads to secondary necrosis, resulting in tissue damage and sustained inflammation through the release of cytotoxic, pro-inflammatory and immunogenic molecules by the lysing cells [13] . Impaired clearance of apoptotic neutrophils is also associated with a variety of inflammatory diseases, including chronic obstructive pulmonary disease (COPD), asthma, pulmonary fibrosis, cystic fibrosis and atherosclerosis, underscoring the importance of this process [14] , [15] , [16] , [17] , [18] , [19] . Macrophages may recognize apoptotic cells for efferocytosis through receptors that bind phosphatidylserine (PS), the ‘eat-me’ signal that is normally localized in the inner leaflet of the plasma membrane and becomes exposed on the outer leaflet of the lipid bilayer on apoptosis. Among known efferocytosis receptors that recognize PS directly are brain-specific angiogenesis inhibitor-1 (BAI-1), Stabilin 1 and 2, and members of the T-cell immunoglobulin mucin domain protein family [11] , [12] . Alternatively, specific factors in serum or produced by macrophages can serve as bridging molecules that bind apoptotic cells via recognition of PS and couple them to macrophages through interaction with various efferocytosis receptors. Known bridging molecules include milk-fat-globule-epidermal growth factor 8 (MFG-E8/Lactaherin) [20] , thrombospondin-1 (ref. 21 ) and protein S/growth arrest-specific gene 6 (Gas6) [22] , [23] , and each recognizes specific efferocytosis receptors on phagocytes including integrins α v β 3 /α v β 5 , CD36 or Tyro3/Axl/Mer (TAM), respectively [12] , [24] . Although the existence of these diverse mechanisms of PS recognition may provide functional redundancy, specific PS recognition molecules or mechanisms may play preferential roles in various organs or contexts, possibly due to their cell-type specificity and time course of the expression [11] , [25] . Despite the importance of neutrophil clearance, no specific bridging molecule or efferocytosis receptor has been identified as key mediators of neutrophil efferocytosis in cutaneous wound healing. One of the proteins whose expression is associated with wound healing is CCN1, a matricellular protein that regulates diverse cellular functions primarily through interaction with distinct integrins in a cell type-specific manner [26] , [27] . CCN1 is organized into four conserved domains with sequence similarities to insulin-like growth factor binding proteins (IGFBP), von Willebrand factor type C repeat (vWC), thrombospondin type 1 repeat (TSR) and a cysteine-knot in the carboxyl terminus (CT). Specific integrin-binding sites have been identified in the vWC, TSR and CT domains [26] , [27] . We have previously shown that CCN1 functions to dampen and resolve fibrosis in wound healing by triggering cellular senescence in myofibroblasts through the engagement of integrin α 6 β 1 via its CT domain during the tissue maturation phase [28] , [29] . Here we show that surprisingly, CCN1 is also indispensable for the clearance of neutrophils, thus serving a distinct function in the early inflammatory phase of wound healing. Mechanistically, it acts as a bridging molecule by binding PS on apoptotic neutrophils through its TSR domain and to integrins α v β 3 /α v β 5 on macrophages through its vWC domain, thereby activating Rac1 in macrophages to trigger efferocytosis. Application of CCN1 protein on slow-healing wounds with persistent neutrophil accumulation, including wounds of diabetic mice, accelerates neutrophil clearance. These findings reveal CCN1 as the key opsonin for neutrophil efferocytosis in cutaneous wound healing, and suggest a potential therapeutic role for CCN1 in certain types of slow-healing wounds. Ccn1 knockdown impedes cutaneous wound healing Our investigation on the role of Ccn1 in cutaneous wound healing uncovered a biphasic pattern of expression in mRNA and protein, with an early peak in the inflammatory phase (day 3) and a late peak in the maturation phase (days 7–9), suggesting distinct functions in these phases ( Fig. 1a,b ). To evaluate this possibility, we applied antisense oligonucleotides (AS-ODN) to excisional cutaneous wounds to knockdown Ccn1 expression ( Fig. 1c ). When wounds were treated with daily administration of Ccn1 AS-ODN from days 3–7 to target the inflammation and tissue formation phases of wound healing, wound closure was delayed with associated robust inflammatory cell accumulation and poor granulation tissue formation ( Fig. 1d,e ). Accumulation of inflammatory cells and impaired granulation tissue formation can be seen when AS-ODN was applied from day 3 to day 5 to target early Ccn 1 expression specifically, but not when applied from day 7 to day 8 to target late expression in the maturation phase ( Supplementary Fig. S1 ), during which CCN1 was previously shown to trigger myofibroblast senescence to restrict fibrosis [28] . These findings indicate that CCN1 may play distinct roles in the early and late phases of wound healing, corresponding to its biphasic expression pattern. 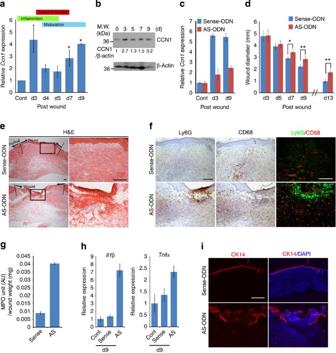Figure 1:Ccn1knockdown impedes healing and neutrophil clearance in cutaneous wounds. (a)Ccn1mRNA levels in cutaneous wound lysates inWTC57BL/6 mice at indicated days post wounding were quantified by qRT–PCR (n=4 per time point). Corresponding phases of wound healing are shown on top. *P<0.008. (b) CCN1 protein in these wounds was analysed by western blotting, and relative CCN1 expression was normalized to β-actin using Image J densitometry. (c)Ccn1mRNA levels in wounds were measured by qRT–PCR after daily application of either sense or antisense oligonucleotide (AS-ODN) from day 1 to day 2 and analysed on day 3, or from days 3 to 7 and analysed on day 9 (n=4 per time point per treatment). (d) Wound diameters were measured on indicated days post wounding in animals treated with sense or AS-ODN from days 3–7 (n=8 per time point per treatment). *P<0.005, **P<0.002. Statistical analyses were conducted using one-sided two-samplet-tests (wound diameter). (e) Wound tissue sections (day 9) were stained with H&E; wound edge was marked with dash lines and area in square box was shown in higher magnification on the right (scale bar, 100 μm). (f) Adjacent wound sections (day 9) were stained with either anti-Ly6G mAb or anti-CD68 polyclonal antibody to visualize neutrophils or macrophages, respectively, and counterstained with haematoxylin. Double immunofluorescence with anti-Ly6G mAb (Green) or anti-CD68 polyclonal antibody (Red) provides contrast for neutrophils and macrophages. Scale bars, 100 μm (g) MPO activity in wounds (day 9) treated with either sense-ODN or AS-ODN (n=4 per treatment). (h) Expression ofIl-1βandTnfαwas measured by qRT–PCR at day 9, normalized tocyclophilin E(n=4 per time point per treatment). (i) Wound sections (day 9) were stained for CK14 (red) to visualize stratified epithelial cells and counterstained with DAPI. Scale bar, 500 μm. qRT–PCR and MPO assay were conducted in triplicates. All data are expressed as mean±s.d. in triplicate determinations. d, day. Figure 1: Ccn1 knockdown impedes healing and neutrophil clearance in cutaneous wounds. ( a ) Ccn1 mRNA levels in cutaneous wound lysates in WT C57BL/6 mice at indicated days post wounding were quantified by qRT–PCR ( n =4 per time point). Corresponding phases of wound healing are shown on top. * P <0.008. ( b ) CCN1 protein in these wounds was analysed by western blotting, and relative CCN1 expression was normalized to β-actin using Image J densitometry. ( c ) Ccn1 mRNA levels in wounds were measured by qRT–PCR after daily application of either sense or antisense oligonucleotide (AS-ODN) from day 1 to day 2 and analysed on day 3, or from days 3 to 7 and analysed on day 9 ( n =4 per time point per treatment). ( d ) Wound diameters were measured on indicated days post wounding in animals treated with sense or AS-ODN from days 3–7 ( n =8 per time point per treatment). * P <0.005, ** P <0.002. Statistical analyses were conducted using one-sided two-sample t -tests (wound diameter). ( e ) Wound tissue sections (day 9) were stained with H&E; wound edge was marked with dash lines and area in square box was shown in higher magnification on the right (scale bar, 100 μm). ( f ) Adjacent wound sections (day 9) were stained with either anti-Ly6G mAb or anti-CD68 polyclonal antibody to visualize neutrophils or macrophages, respectively, and counterstained with haematoxylin. Double immunofluorescence with anti-Ly6G mAb (Green) or anti-CD68 polyclonal antibody (Red) provides contrast for neutrophils and macrophages. Scale bars, 100 μm ( g ) MPO activity in wounds (day 9) treated with either sense-ODN or AS-ODN ( n =4 per treatment). ( h ) Expression of Il-1β and Tnfα was measured by qRT–PCR at day 9, normalized to cyclophilin E ( n =4 per time point per treatment). ( i ) Wound sections (day 9) were stained for CK14 (red) to visualize stratified epithelial cells and counterstained with DAPI. Scale bar, 500 μm. qRT–PCR and MPO assay were conducted in triplicates. All data are expressed as mean±s.d. in triplicate determinations. d, day. Full size image In sense-ODN-treated control wounds, resolution of inflammation, formation of granulation tissue and re-epithelialization were observed within a 9-day period ( Fig. 1d–f,i ). By contrast, immunohistochemical and double immunofluorescence staining of AS-ODN-treated wounds for neutrophils and macrophages with anti-Ly6G and CD68 antibodies, respectively, revealed an aberrant and exuberant accumulation of neutrophils ( Fig. 1f and Supplementary Fig. S2 ). Myeloperoxidase (MPO) activity was >4-fold higher in AS-ODN-treated wounds than sense-ODN-treated controls, confirming a large accumulation of neutrophils ( Fig. 1g ). Consistently, the pro-inflammatory cytokines Il-1β and Tnfα were expressed at 7- and 2.3-fold higher levels in AS-ODN-treated wounds, respectively ( Fig. 1h ). Neutrophils and macrophages are major cell types expressing CCN1 in the wounds during the inflammatory phase as judged by the co-localization of CCN1 with these immune cells, and AS-ODN effectively eliminated CCN1 protein expression in these cells ( Supplementary Fig. S3 ). Consistent with the accumulation of neutrophils and the short lifespan of these cells, enhanced accumulation of apoptotic cells was observed in AS-ODN-treated wounds ( Supplementary Fig. S4 ). Moreover, AS-ODN-treated wounds exhibited impaired re-epithelialization as shown by immunostaining of the stratified epithelial cell marker cytokeratin 14 (CK14; Fig. 1i ). However, CCN1 does not have a direct effect on keratinocyte migration ( Supplementary Fig. S5 ), suggesting that impaired re-epithelialization is secondary to other defects in these wounds. Together these results indicate that Ccn1 knockdown leads to neutrophil persistence and delayed wound healing, suggesting that wounds deficient in CCN1 function are stalled at the inflammatory phase. Impaired skin wound healing in Ccn1 D125A/D125A knockin mice CCN1 exerts diverse effects on cellular functions primarily through direct binding to distinct integrins in a cell type-specific manner [26] . To dissect CCN1 functions through distinct integrin receptor pathways, we examined knockin mice expressing mutant CCN1 unable to bind specific integrins. For example, Ccn1 DM/DM mice carry mutations in the overlapping binding sites for integrin α 6 β 1 , the major CCN1 receptor in fibroblastic cells [30] , and integrin α M β 2 , the adhesion receptor for monocytes [31] . However, Ccn1 DM/DM knockin mice did not exhibit any observable inflammatory phenotype, but showed exacerbated fibrosis due to the inability to activate α 6 β 1 in fibroblasts [28] . Although lacking an RGD sequence, CCN1 binds integrins α v β 3 and α v β 5 through a non-canonical site in its vWC domain [32] . To assess the role of CCN1 mediated through α v integrins, we constructed knockin mice in which the Ccn1 genomic locus was replaced by Ccn1 D125A ( Fig. 2a ), a mutant allele encoding a single amino-acid substitution (Asp-125 to Ala) that abolished CCN1 binding to α v integrins [32] . Knockin of the mutant allele was confirmed by standard molecular methods including direct sequencing, and illustrated by the presence of the predicted PCR products ( Fig. 2b ). Whereas Ccn1 -null mice are embryonic lethal due to cardiovascular defects [33] , [34] , Ccn1 D125A/D125A mice are viable, fertile and exhibit no apparent abnormalities, indicating the CCN1-D125A mutant protein is biologically active and does not impair essential functions during development. 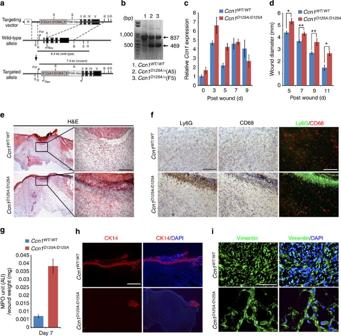Figure 2:Ccn1D125A/D125Aknockin mice phenocopy mice withCcn1knockdown in wound healing. (a) Construction ofCcn1D125A/+knockin mice. A gene targeting construct has the EcoRI–XmaI fragment ofCcn1replaced with cDNA encoding CCN1-D125A. The recombinant allele maintained theCcn1promoter and transcription start site and expresses theCcn1D125AcDNA preserving theCcn15′ and 3′ untranslated sequences. Thymidine kinase (tk) and PGK-neowere used as selectable markers in homologous recombination in ES cells. B,BamHI; X,XmaI; R,EcoRI; S,SphI; for, forward primer; rev, reverse primer. (b) DNA isolated fromCcn1WT/WT(WT) mice and two separate ES clones (A5 and F5) ofCcn1D125A/+mice were PCR-amplified, yielding 837 bp (WT) and 469 bp (targeted) bands. (c)Ccn1mRNA expression in WT andCcn1D125A/D125Amice was quantified using qRT–PCR and normalized tocyclophilin E(n=4 per time point per genotype). (d) Wound diameters were measured inWTorCcn1D125A/D125Amice at indicated days post wounding (n=8 per time point per genotype). *P<0.002, **P<0.0005. (e) Wound sections (day 7) were stained with H&E. Area in square box was visualized under higher magnification on the right. Scale bars, 100 μm. (f) Adjacent sections were stained with anti-Ly6G or anti-CD68. Double immunofluorescence staining of Ly6G (green) and CD68 (red) was shown on the right (scale bar, 100 μm). (g) MPO activity in day 7 wounds ofWTorCcn1D125A/D125Amice was measured (n=4 for each genotype). Wound sections were stained for either (h) CK14 (red; scale bar, 500 μm) or (i) vimentin (green; scale bar, 50 μm) and visualized under immunofluorescence, and counterstained with DAPI (blue). Statistical analyses were conducted using one-sided two-samplet-tests (wound diameter). qRT–PCR and MPO assay are expressed as mean±s.d. in triplicate determinations. Figure 2: Ccn1 D125A/D125A knockin mice phenocopy mice with Ccn1 knockdown in wound healing. ( a ) Construction of Ccn1 D125A/+ knockin mice. A gene targeting construct has the EcoRI–XmaI fragment of Ccn1 replaced with cDNA encoding CCN1-D125A. The recombinant allele maintained the Ccn1 promoter and transcription start site and expresses the Ccn1 D125A cDNA preserving the Ccn1 5′ and 3′ untranslated sequences. Thymidine kinase (tk) and PGK- neo were used as selectable markers in homologous recombination in ES cells. B, Bam HI; X, Xma I; R, Eco RI; S, Sph I; for, forward primer; rev, reverse primer. ( b ) DNA isolated from Ccn1 WT/WT ( WT ) mice and two separate ES clones (A5 and F5) of Ccn1 D125A/+ mice were PCR-amplified, yielding 837 bp (WT) and 469 bp (targeted) bands. ( c ) Ccn1 mRNA expression in WT and Ccn1 D125A/D125A mice was quantified using qRT–PCR and normalized to cyclophilin E ( n =4 per time point per genotype). ( d ) Wound diameters were measured in WT or Ccn1 D125A/D125 A mice at indicated days post wounding ( n =8 per time point per genotype). * P <0.002, ** P <0.0005. ( e ) Wound sections (day 7) were stained with H&E. Area in square box was visualized under higher magnification on the right. Scale bars, 100 μm. ( f ) Adjacent sections were stained with anti-Ly6G or anti-CD68. Double immunofluorescence staining of Ly6G (green) and CD68 (red) was shown on the right (scale bar, 100 μm). ( g ) MPO activity in day 7 wounds of WT or Ccn1 D125A/D125 A mice was measured ( n =4 for each genotype). Wound sections were stained for either ( h ) CK14 (red; scale bar, 500 μm) or ( i ) vimentin (green; scale bar, 50 μm) and visualized under immunofluorescence, and counterstained with DAPI (blue). Statistical analyses were conducted using one-sided two-sample t -tests (wound diameter). qRT–PCR and MPO assay are expressed as mean±s.d. in triplicate determinations. Full size image Expression of mutant Ccn1 is elevated in cutaneous wounds in Ccn1 D125A/D125A mice, similar to wild-type (WT) mice ( Fig. 2c ). Ccn1 D125A/D125A mice experienced significantly slower cutaneous wound closure than WT mice, with poor granulation tissue formation and aberrant accumulation of inflammatory cells similar to the effects of Ccn1 knockdown ( Fig. 2d,e ). Immunostaining for Ly6G and CD68 and double immunofluorescence showed that neutrophils were accumulated in wounds of Ccn1 D125A/D125A mice ( Fig. 2f ), and this result was confirmed by MPO assay ( Fig. 2g ). Moreover, immunostaining for CK14 and vimentin indicated that re-epithelialization and granulation tissue formation, respectively, were impaired ( Fig. 2h,i ). As CCN1 is known to induce angiogenesis through α v β 3 (refs 35 , 36 ), we examined angiogenesis in wounds of Ccn1 D125A/D125A mice. Indeed, these mice exhibited reduced numbers of CD31-positive endothelial cells and blood vessels, fewer vessel-associated mural cells or pericytes as judged by staining for NG2 and desmin, as well as diminished expression of angiogenic growth factors ( Supplementary Fig. S6 ). Since the α 6 β 1 -binding site required for CCN1 induction of myofibroblast senescence was not affected by the D125A mutation [28] , senescence occurred successfully in wounds of Ccn1 D125A/D125A mice ( Supplementary Fig. S7a ). However, collagen deposition and tissue maturation was delayed, peaking at day 11 instead of day 9 in WT, consistent with delayed healing in these mice ( Supplementary Fig. S7b ). The phenotypes of Ccn1 D125A/D125A mice closely resemble the effects of Ccn1 knockdown, suggesting that critical CCN1 functions in the inflammatory phase of wound healing are mediated through α v integrins. Neutrophil depletion accelerates repair in Ccn1 knockin mice Consistent with increased neutrophil accumulation in Ccn1 D125A/D125A wounds, elevated expression of the pro-inflammatory cytokines Tnfα and Il-1β was observed ( Fig. 3a,b ). Expression of the neutrophil chemoattractants Cxcl1 (KC, GROα) and Cxcl5 (LIX), as well as their receptor Cxcr2 , was elevated and more sustained in Ccn1 D125A/D125A wounds ( Fig. 3c–e ), suggesting that there may be enhanced recruitment of neutrophils to the wound site. Since macrophages in wounds are mostly derived from monocytes recruited from circulation, the elevated and sustained expression of Ccl2 encoding the monocyte chemotactic protein-1 was also consistent with increases in macrophages ( Fig. 3f ). These cytokine expression patterns may be due to aberrant recruitment of, or gene expression by, inflammatory cells, or alternatively, impaired neutrophil apoptosis or clearance [6] . However, there was no difference in the number of neutrophils in the peripheral blood of WT and Ccn1 D125A/D125A mice ( Fig. 4a ), suggesting no disparity in the systemic level of neutrophil production and mobilization. The expression of granulocyte colony-stimulating factor ( Gcsf ) in the wounds was also similar ( Supplementary Fig. S8 ). Moreover, CCN1 protein had no effect on apoptosis of bone marrow-derived neutrophils ( Supplementary Fig. S9 ), and there was no defect in Ccn1 D125A/D125A macrophage gene expression when exposed to M1- or M2-polarizing agents ( Supplementary Fig. S10 ). Together, these results indicate that neutrophil accumulation in Ccn1 D125A/D125A mice is not likely due to aberrant production, mobilization or apoptosis of neutrophils, nor deranged gene expression in macrophages. 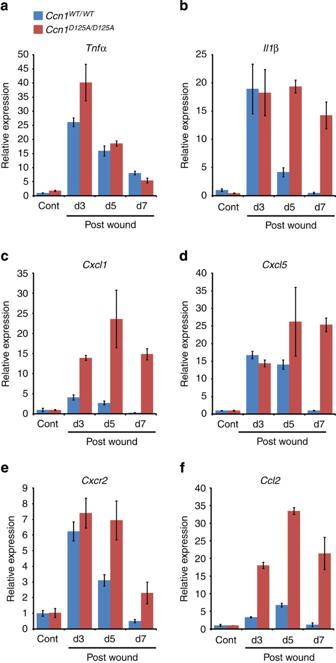Figure 3: Sustained expression of chemokines and cytokines inCcn1D125A/D125Awounds. Expression of various cytokines, chemokines and chemokine receptors in WT andCcn1D125A/D125Amice was measured by qRT–PCR, normalized tocyclophilin E(n=3 per time point per genotype). (a)Tnfα. (b)Il-1β. (c)Cxcl1(KC/Groα). (d)Cxcl5(LIX). (e)Cxcr2.(f)Ccl2(MCP-1). Data represent mean±s.d. in triplicate determinations. d, day. Figure 3: Sustained expression of chemokines and cytokines in Ccn1 D125A/D125A wounds. Expression of various cytokines, chemokines and chemokine receptors in WT and Ccn1 D125A/D125A mice was measured by qRT–PCR, normalized to cyclophilin E ( n =3 per time point per genotype). ( a ) Tnfα . ( b ) Il-1β . ( c ) Cxcl1 ( KC/Groα ). ( d ) Cxcl5 ( LIX ). ( e ) Cxcr2. ( f ) Ccl2 ( MCP-1 ). Data represent mean±s.d. in triplicate determinations. d, day. 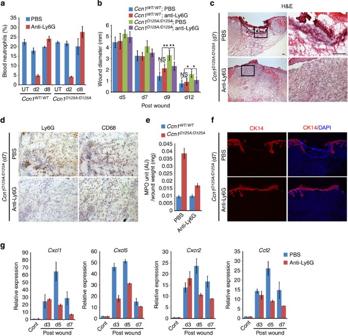Figure 4: Neutrophil depletion accelerates wound healing inCcn1D125A/D125Amice. (a) A single i.p. injection of anti-Ly6G mAb was delivered 1 day before wounding, and the neutrophil levels were measured by complete blood count at indicated days after wounding (n=6 for time point per treatment). Untreated (UT) mice were used as control (n=3 per genotype). (b) Wound diameters were measured in WT andCcn1D125A/D125Amice treated with anti-Ly6G mAb or PBS control (n=8 per data point). NS,P>0.05; *P<0.001, **P<0.0001 in one-sided two-samplet-tests and analysis of variance with Bonferronipost hoctests. (c) Wound tissues (day 7) from mice treated with anti-Ly6G mAb or PBS were stained with H&E; area in box was enlarged on the right. Scale bar, 100 μm. (d) Adjacent sections were stained with either anti-Ly6G or anti-CD68 and counterstained with hematoxylin (scale bar, 100 μm). Ly6G-positive neutrophils are greatly reduced after neutrophil depletion. (e) MPO activity was measured in day 7 wounds of mice treated with anti-Ly6G mAb or PBS (n=4 per data point). (f) Immunofluorescence staining of CK14 (red) in day 7 wounds ofCcn1D125A/D125Amice treated with either PBS or anti-Ly6G and counterstained with DAPI (blue). Scale bar, 500 μm. (g) Expression of chemokines (Cxcl1,Cxcl5andCcl2) and chemokine receptor (Cxcr2) in wounds ofCcn1D125A/D125Amice treated with either anti-Ly6G mAb or PBS was measured by qRT–PCR and normalized tocyclophilin E(n=4 per data point). Data are expressed as mean±s.d. in triplicate determinations. d, day. Full size image Figure 4: Neutrophil depletion accelerates wound healing in Ccn1 D125A/D125A mice. ( a ) A single i.p. injection of anti-Ly6G mAb was delivered 1 day before wounding, and the neutrophil levels were measured by complete blood count at indicated days after wounding ( n =6 for time point per treatment). Untreated (UT) mice were used as control ( n =3 per genotype). ( b ) Wound diameters were measured in WT and Ccn1 D125A/D125A mice treated with anti-Ly6G mAb or PBS control ( n =8 per data point). NS, P >0.05; * P <0.001, ** P <0.0001 in one-sided two-sample t -tests and analysis of variance with Bonferroni post hoc tests. ( c ) Wound tissues (day 7) from mice treated with anti-Ly6G mAb or PBS were stained with H&E; area in box was enlarged on the right. Scale bar, 100 μm. ( d ) Adjacent sections were stained with either anti-Ly6G or anti-CD68 and counterstained with hematoxylin (scale bar, 100 μm). Ly6G-positive neutrophils are greatly reduced after neutrophil depletion. ( e ) MPO activity was measured in day 7 wounds of mice treated with anti-Ly6G mAb or PBS ( n =4 per data point). ( f ) Immunofluorescence staining of CK14 (red) in day 7 wounds of Ccn1 D125A/D125A mice treated with either PBS or anti-Ly6G and counterstained with DAPI (blue). Scale bar, 500 μm. ( g ) Expression of chemokines ( Cxcl1 , Cxcl5 and Ccl2 ) and chemokine receptor ( Cxcr2 ) in wounds of Ccn1 D125A/D125A mice treated with either anti-Ly6G mAb or PBS was measured by qRT–PCR and normalized to cyclophilin E ( n =4 per data point). Data are expressed as mean±s.d. in triplicate determinations. d, day. Full size image It was observed that the deletion of macrophages in the inflammatory phase of wound healing led to vascularization defect, reduced granulation tissue formation and impaired re-epithelialization, similar to aspects of the Ccn1 D125A/D125A phenotype [37] . Since deletion of macrophages may lead to impaired neutrophil clearance, we tested the hypothesis that neutrophil persistence may be the cause of wound-healing defects in Ccn1 D125A/D125A mice by depleting neutrophils using a well-characterized monoclonal antibody (mAb) against Ly6G (RB6-8C5) [38] . Previous studies showed that neutrophil depletion during wound healing either had no effect or accelerated re-epithelialization [39] , [40] . A single intraperitoneal (i.p.) injection of anti-Ly6G mAb 1 day before wounding decreased neutrophils from ∼ 15–20% of blood cells to <4% by day 2 post wounding in both WT and Ccn1 D125A/D125A mice; thereafter, neutrophils recovered to the normal level by day 8 ( Fig. 4a ) [40] . In WT mice, wound closure was unaffected by anti-Ly6G mAb treatment up to day 7 but was slightly retarded by day 9, although the difference did not reach statistical significance ( P >0.05; Fig. 4b ). By contrast, neutrophil depletion accelerated wound closure in Ccn1 D125A/D125A mice to essentially the same rate as similarly treated WT mice (* P <0.001; ** P <0.0001; Fig. 4b ). Anti-Ly6G mAb-treated Ccn1 D125A/D125A wounds showed much reduced neutrophil accumulation and improved granulation tissue formation as judged by staining with haematoxylin and eosin (H&E) and immunostaining for Ly6G and CD68 ( Fig. 4c,d ). MPO assay also confirmed reduction of neutrophils in day 7 wounds ( Fig. 4e ). Moreover, neutrophil depletion in Ccn1 D125A/D125A mice resulted in greatly improved re-epithelialization, as evidenced by CK14 staining ( Fig. 4f ). Concomitantly, substantial reduction in the expression of the monocyte chemokine Ccl2 as well as the neutrophil chemokines Cxcl1 and Cxcl5 and their receptor Cxcr2 was also observed ( Fig. 4g ). Thus, neutrophil depletion accelerated wound closure and rectified many of the wound healing-associated defects in Ccn1 D125A/D125A mice, indicating that neutrophil persistence is the underlying cause of elevated chemokine expression, impaired granulation tissue formation, and delayed wound healing in Ccn1 D125A/D125A mice. CCN1 mediates neutrophil efferocytosis through α v integrins Since integrin α v β 3 is known to function as an efferocytosis receptor on macrophages [21] , we hypothesized that CCN1 might regulate phagocytosis of apoptotic neutrophils by macrophages through α v integrins. To evaluate this possibility, we harvested neutrophils and macrophages from bone marrow of WT and Ccn1 D125A/D125A mice ( Supplementary Figs S9 and S10 ). When WT macrophages (labelled with CellTracker Green CMFDA) were incubated with aged WT neutrophils (labelled blue with 4′,6-diamidino-2-phenylindole (DAPI)), efferocytosis was evident with multiple neutrophils detected inside macrophages ( Fig. 5a ). However, WT neutrophils were inefficiently engulfed by macrophages from Ccn1 D125A/D125A mice, indicating a role for CCN1 in efferocytosis ( Fig. 5a ). Efferocytosis was substantially diminished when either neutrophils or macrophages were from Ccn1 D125A/D125A mice, and further reduced when both neutrophils and macrophages were from these mice. These results indicate that CCN1 functions to regulate both cell types in efferocytosis in a non-cell-autonomous manner ( Fig. 5b ). 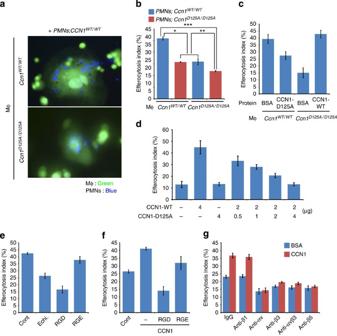Figure 5: CCN1 mediates efferocytosis through integrins αvβ3/αvβ5. Neutrophils (PMNs) and macrophages (MΦ) were isolated from bone marrow of WT andCcn1D125A/D125Amice. Aged apoptotic neutrophils (labelled blue with DAPI, 10 mg ml−1) were incubated with macrophages (labelled green with CellTracker green, 5 μM) for 60 min and number of DAPI-positive macrophages were counted under fluorescence microscopy and expressed as percentages of total macrophages. (a) Representative images showing WT neutrophils (blue) were abundantly engulfed by WT macrophages (Green), whereas few were visible in macrophages isolated fromCcn1D125A/D125Amice. Scale bar, 40 μm. (b) Neutrophils and macrophages from WT orCcn1D125A/D125Amice were incubated in various combinations as indicated for 90 min. Reduced efferocytosis was observed when either neutrophils or macrophages were fromCcn1D125A/D125Amice (n=3 per group). *P<0.005, **P<0.0005, ***P<0.00005 in one-sided two-samplet-tests and analysis of variance with Bonferronipost hoctests. (c) Neutrophils (WT) were pretreated with bovine serum albumin (BSA; control), CCN1-WT or CCN1-D125A mutant protein (4 μg ml−1) for 60 min, and incubated with macrophages from eitherWTorCcn1D125A/D125Amice for efferocytosis (n=3 per group). (d) Neutrophils (WT) were pretreated with either CCN1-WT, CCN1-D125A protein individually or CCN1-WT protein with increasing amounts of CCN1-D125A for 60 min, followed by incubation with macrophages (WT) for 60 min to evaluate the dominant-negative effect of CCN1-D125A (n=3 per group) (e) WT macrophages were pretreated for 30 min with integrin antagonists Echistatin (10 nM), RGD peptide (20 μM) or RGE peptide (20 μM) and WT neutrophils were then added and incubated for 90 min (n=3 per group). (f) WT macrophages were preloaded with RGD or RGE as above, and incubated with WT neutrophils with CCN1 for efferocytosis (n=3 per group). Incubation time was reduced to 60 min. (g) WT macrophages were pretreated with function-blocking mAbs against indicated integrins (50 μg ml−1; each) and efferocytosis of WT neutrophils treated with PBS or CCN1 was measured (n=3 per group). All data are expressed as mean±s.d. in triplicate determinations. Figure 5: CCN1 mediates efferocytosis through integrins α v β 3 /α v β 5 . Neutrophils (PMNs) and macrophages (MΦ) were isolated from bone marrow of WT and Ccn1 D125A/D125A mice. Aged apoptotic neutrophils (labelled blue with DAPI, 10 mg ml −1 ) were incubated with macrophages (labelled green with CellTracker green, 5 μM) for 60 min and number of DAPI-positive macrophages were counted under fluorescence microscopy and expressed as percentages of total macrophages. ( a ) Representative images showing WT neutrophils (blue) were abundantly engulfed by WT macrophages (Green), whereas few were visible in macrophages isolated from Ccn1 D125A/D125A mice. Scale bar, 40 μm. ( b ) Neutrophils and macrophages from WT or Ccn1 D125A/D125A mice were incubated in various combinations as indicated for 90 min. Reduced efferocytosis was observed when either neutrophils or macrophages were from Ccn1 D125A/D125A mice ( n =3 per group). * P <0.005, ** P <0.0005, *** P <0.00005 in one-sided two-sample t -tests and analysis of variance with Bonferroni post hoc tests. ( c ) Neutrophils (WT) were pretreated with bovine serum albumin (BSA; control), CCN1-WT or CCN1-D125A mutant protein (4 μg ml −1 ) for 60 min, and incubated with macrophages from either WT or Ccn1 D125A/D125A mice for efferocytosis ( n =3 per group). ( d ) Neutrophils (WT) were pretreated with either CCN1-WT, CCN1-D125A protein individually or CCN1-WT protein with increasing amounts of CCN1-D125A for 60 min, followed by incubation with macrophages ( WT ) for 60 min to evaluate the dominant-negative effect of CCN1-D125A ( n =3 per group) ( e ) WT macrophages were pretreated for 30 min with integrin antagonists Echistatin (10 nM), RGD peptide (20 μM) or RGE peptide (20 μM) and WT neutrophils were then added and incubated for 90 min ( n =3 per group). ( f ) WT macrophages were preloaded with RGD or RGE as above, and incubated with WT neutrophils with CCN1 for efferocytosis ( n =3 per group). Incubation time was reduced to 60 min. ( g ) WT macrophages were pretreated with function-blocking mAbs against indicated integrins (50 μg ml −1 ; each) and efferocytosis of WT neutrophils treated with PBS or CCN1 was measured ( n =3 per group). All data are expressed as mean±s.d. in triplicate determinations. Full size image Next, we examined the effect of exogenously added CCN1 protein on efferocytosis ( Fig. 5c ). WT CCN1 protein was able to restore efferocytosis in Ccn1 D125A/D125A macrophages to WT levels, showing that CCN1 can directly promote efferocytosis. However, the CCN1-D125A mutant protein inhibited efferocytosis in WT macrophages ( Fig. 5c ), suggesting that it might be able to act in a dominant-negative manner. Indeed, addition of an increasing amount of CCN1-D125A protein progressively inhibited the stimulatory effect of WT CCN1 on efferocytosis, showing dominant-negative action ( Fig. 5d ). This observation may help to explain the reduced efferocytsis observed when either neutrophils or macrophages were isolated from Ccn1 D125A/D125A mice ( Fig. 5b ), since the mutant CCN1 protein inhibits WT CCN1 function. Blocking α v integrins with known antagonists such as echistatin or RGD peptide inhibited efferocytosis, whereas the RGE control peptide had no effect ( Fig. 5e ). Inhibition by RGD peptide was observed even in the presence of exogenously added CCN1 protein, consistent with α v integrins acting downstream of CCN1 ( Fig. 5f ). Furthermore, macrophages pretreated with function-blocking mAbs against integrins α v , β 3 , β 5 and α v β 3 abrogated CCN1-stimulated efferocytosis, whereas IgG control or anti-β 1 mAb had no effect ( Fig. 5g ). Together with the loss of efferocytosis activity in the D125A mutant, these results establish that CCN1 acts through integrins α v β 3 and α v β 5 . Phagocytosis requires cytoskeletal reorganization and movement to form phagosomes, a process dependent on the activation of the small GTPase Rac1 (ref. 24 ). Activation of α v β 5 is thought to trigger the recruitment of the p130 Cas /CrkII/Dock180 complex, which activates Rac1 and promotes efferocytosis [41] . We found that CCN1 stimulated the formation of the p130 Cas /CrkII complex in macrophages, as shown by reciprocal co-immunoprecipitation ( Fig. 6a,b ). Tyrosine phosphorylation of the focal adhesion kinase (FAK) was also dependent on the formation this p130 Cas /CrkII signalling complex [42] , which occurred in a CCN1-dependent manner ( Fig. 6c ). Furthermore, we demonstrate that CCN1 induced the activation of Rac1 in bone marrow-derived macrophages ( Fig. 6d ). CCN1-induced formation of the p130 Cas /CrkII signalling complex, FAK phosphorylation and activation of Rac1 are each dependent on CCN1 interaction with α v β 3 /α v β 5 , as they were abolished in the D125A mutant ( Fig. 6 ). 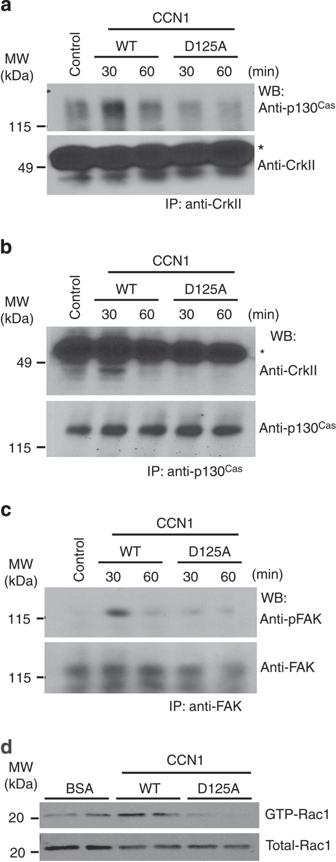Figure 6: CCN1 activates Rac1 and p130Cas-CrkII complex formation in murine macrophages. (a) Raw264.7 murine macrophages were either untreated (Control) or treated with either CCN1-WT or CCN1-D125A proteins for indicated times and complex formation was analysed by immunoprecipitation (IP) with anti-CrkII antibodies followed by immunoblotting with anti-p130Casantibodies. The same lysates were further analysed by IP with anti-p130Casantibodies followed by immunoblotting with anti-CrkII antibodies (b). (c) FAK activation was analysed with IP and western blotting: IP with anti-FAK and WB with anti-phosphoFAK. *(asterisk) is immunoglobulin heavy chain. (d) Rac1 activation in bone marrow-derived macrophages (Ccn1WT/WT) was evaluated after treatment with bovine serum albumin (BSA), CCN1-WT or CCN1-D125A mutant proteins (4 μg ml−1) for 60 min using PAK-PBD agarose (20 μg for each sample) pull-down assay. Total lysates were used to verify total Rac1 expression by immunoblotting (lower panel). Figure 6: CCN1 activates Rac1 and p130 Cas -CrkII complex formation in murine macrophages. ( a ) Raw264.7 murine macrophages were either untreated (Control) or treated with either CCN1-WT or CCN1-D125A proteins for indicated times and complex formation was analysed by immunoprecipitation (IP) with anti-CrkII antibodies followed by immunoblotting with anti-p130 Cas antibodies. The same lysates were further analysed by IP with anti-p130 Cas antibodies followed by immunoblotting with anti-CrkII antibodies ( b ). ( c ) FAK activation was analysed with IP and western blotting: IP with anti-FAK and WB with anti-phosphoFAK. *(asterisk) is immunoglobulin heavy chain. ( d ) Rac1 activation in bone marrow-derived macrophages ( Ccn1 WT/WT ) was evaluated after treatment with bovine serum albumin (BSA), CCN1-WT or CCN1-D125A mutant proteins (4 μg ml −1 ) for 60 min using PAK-PBD agarose (20 μg for each sample) pull-down assay. Total lysates were used to verify total Rac1 expression by immunoblotting (lower panel). Full size image CCN1 functions as a bridging molecule As phagocytic receptors on macrophages, integrins α v β 3 and α v β 5 do not directly recognize the so called ‘eat-me’ signals, such as PS, on apoptotic cells. Instead, a molecule that can bind both PS and the integrins is required to bridge the apoptotic cells to α v β 3 /α v β 5 on macrophages [10] . To test whether CCN1 may act as a bridging molecule, we first examined its ability to bind PS directly using solid-phase enzyme-linked immunosorbent assay. We found that PS efficiently bound to CCN1-WT protein as well as to the CCN1-D125A [32] (unable to bind α v β 3 /α v β 5 ) and CCN1-DM [30] (unable to bind α 6 β 1 /α M β 2 ) with half maximal binding occurring at ∼ 20–25 nM CCN1, but not to laminin ( Fig. 7a ). Although laminin was previously shown to bind to glycolipids and phospholipids, it required a much higher concentration (>10 μg) of lipids for binding [43] . To confirm that CCN1 binding to PS mediates its function in efferocytosis, PS-containing liposomes were used as competitive inhibitors ( Fig. 7b ). Although exogenously added CCN1 protein enhanced efferocytosis, its effect was strongly inhibited when CCN1 was preloaded with PS-liposomes, indicating that CCN1 binding to PS is critical for its bridging function. 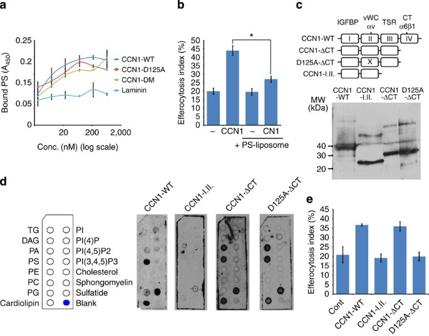Figure 7: CCN1 functions as a bridging molecule by direct binding to PS through its TSR domain. (a) CCN1 binding to PS was assessed by solid-phase enzyme-linked immunosorbent assay. Serial dilution of recombinant CCN1 proteins (WT, D125A or DM mutants) or Laminin were precoated on to 96-well plate and blocked with bovine serum albumin (BSA; 10 mg ml−1). After PS (300 ng per well) was added and incubated for 1 h, bound-PS was detected by anti-PS mAb (1 μg per well). Coated proteins were plotted with logarithmic scale (n=3 per each concentration) (b) Efferocytosis assay was performed using WT neutrophils and macrophages. Where indicated, CCN1 protein alone or preincubated with liposomes containing phospho-L-Serine was added to the assay (n=4 per treatment). *P<0.001 in one-sided two-samplet-tests. (c) Schematic diagram of CCN1 deletion mutants (top). Purified deletion mutant proteins were confirmed by immunoblotting using polyclonal anti-CCN1 vWC domain antibodies (bottom). (d) Binding of CCN1 and mutant proteins to membranes spotted with phospholipids (DAG, diacylglycerol; PC, phosphatidylcholine; PE, phosphatidylethanolamine; PG, phosphatidylglycerol; PI, phosphatidylinositol; PI(4)P, phosphatidylinositol-4-phosphate; PI(4,5)P2, phosphatidylinositol-4,5-biphosphate; PI(3,4,5)P3, phosphatidylinositol-3,4,5-triphosphate; TG, triglycerol). Proteins (10 μg each) were incubated with the membranes and bound proteins detected by immunoblotting with anti-vWC antibodies. Representative results from triplicate experiments are shown. (e) Purified recombinant CCN1 proteins (WT and deletion mutants) were preincubated with aged neutrophils and efferocytosis was measured (n=4 per treatment). Data expressed as mean±s.d. in triplicate determinations. Figure 7: CCN1 functions as a bridging molecule by direct binding to PS through its TSR domain. ( a ) CCN1 binding to PS was assessed by solid-phase enzyme-linked immunosorbent assay. Serial dilution of recombinant CCN1 proteins (WT, D125A or DM mutants) or Laminin were precoated on to 96-well plate and blocked with bovine serum albumin (BSA; 10 mg ml −1 ). After PS (300 ng per well) was added and incubated for 1 h, bound-PS was detected by anti-PS mAb (1 μg per well). Coated proteins were plotted with logarithmic scale ( n =3 per each concentration) ( b ) Efferocytosis assay was performed using WT neutrophils and macrophages. Where indicated, CCN1 protein alone or preincubated with liposomes containing phospho- L -Serine was added to the assay ( n =4 per treatment). * P <0.001 in one-sided two-sample t -tests. ( c ) Schematic diagram of CCN1 deletion mutants (top). Purified deletion mutant proteins were confirmed by immunoblotting using polyclonal anti-CCN1 vWC domain antibodies (bottom). ( d ) Binding of CCN1 and mutant proteins to membranes spotted with phospholipids (DAG, diacylglycerol; PC, phosphatidylcholine; PE, phosphatidylethanolamine; PG, phosphatidylglycerol; PI, phosphatidylinositol; PI(4)P, phosphatidylinositol-4-phosphate; PI(4,5)P2, phosphatidylinositol-4,5-biphosphate; PI(3,4,5)P3, phosphatidylinositol-3,4,5-triphosphate; TG, triglycerol). Proteins (10 μg each) were incubated with the membranes and bound proteins detected by immunoblotting with anti-vWC antibodies. Representative results from triplicate experiments are shown. ( e ) Purified recombinant CCN1 proteins (WT and deletion mutants) were preincubated with aged neutrophils and efferocytosis was measured ( n =4 per treatment). Data expressed as mean±s.d. in triplicate determinations. Full size image CCN1 contains a thrombospondin type I repeat (TSR) in its third domain ( Fig. 7c ). As the TSR motif in BAI-1 can bind PS [44] , we tested whether CCN1 binding to PS is mediated through its TSR. For this purpose, several deletion mutants were constructed ( Fig. 7c ) and the binding of purified deletion mutant proteins to PS was tested using membranes on which various phospholipids were spotted ( Fig. 7d ). Bound CCN1 was detected using anti-CCN1 vWC domain antibodies, which recognized all deletion mutants equally ( Fig. 7c ). Consistent with the solid-phase binding assay above, CCN1 showed strong binding to PS, but not to other negatively charged lipids. It also bound to the mitochondrial inner membrane lipid cardiolipin and sulfatide, as observed for the TSR of BAI-1 (ref. 44 ). Both CCN1-ΔCT and D125A-ΔCT proteins were also capable of binding to PS, cardiolipin and sulfatide, indicating that the C-terminal domain (CT) of CCN1 is dispensable for PS binding. These deletion mutants also bound phosphatidic acid (PA), which was not recognized by full-length CCN1, suggesting that removal of the CT domain may reveal a cryptic binding site for PA in TSR. By contrast, CCN1-I.II, which is lacking both the TSR and CT domains, did not bind to any lipid on the strip, indicating that CCN1 binding to PS requires the TSR domain ( Fig. 7d ). Since the mutant protein CCN1-I.II does not bind PS and the D125A-ΔCT does not bind integrins α v β 3 /α v β 5 , these mutant proteins did not stimulate neutrophil efferocytosis ( Fig. 7e ). By contrast, CCN1-WT and CCN1-ΔCT, being able to bind both PS and integrins α v β 3 /α v β 5 , enhanced neutrophils efferocytosis by macrophages ( Fig. 7e ). Together, these results show that CCN1 is a novel opsonin molecule for efferocytosis by bridging apoptotic neutrophils to macrophages through direct interaction with PS and integrins α v β 3 /α v β 5 , leading to the activation of Rac1 and phagocytosis. CCN1 accelerates neutrophil clearance in slow-healing wounds In view of the activity of CCN1 in efferocytosis, we tested its ability to accelerate neutrophil clearance in slow-healing wounds. A single dose of recombinant WT CCN1 protein or vehicle (PBS) was applied to wounds of Ccn1 D125A/D125A mice at day 6 post wounding and wounds were analysed 1 day later ( Fig. 8a ). H&E staining showed high neutrophil accumulation in PBS-treated Ccn1 D125A/D125A mice, whereas the number of neutrophils significantly decreased in CCN1-treated mice with proportionately more associated macrophages ( Fig. 8a ). MPO assays confirmed that the treatment of wounds with WT CCN1 significantly reduced neutrophils in Ccn1 D125A/D125A mice, whereas treatment with CCN1-D125A protein had no effect ( Fig. 8b ). Moreover, expression of the pro-inflammatory cytokine Il-1β was reduced on treatment with CCN1 protein in Ccn1 D125A/D125A mice, consistent with curtailed inflammation ( Fig. 8c ). 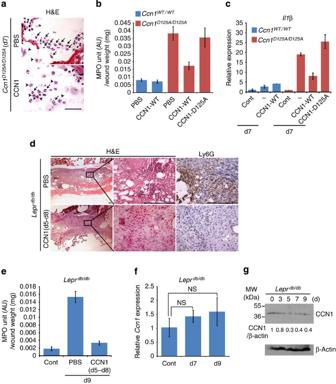Figure 8: CCN1 accelerates neutrophil clearance in slow-healing wounds. (a) Wounds ofCcn1D125A/D125Amice were treated with recombinant WT CCN1 protein (0.2 mg ml−1, 50 μl per dose) or PBS at day 6 and wound tissues were harvested at day 7, sectioned and stained with H&E. (n=4 per treatment). Representative images were shown. Arrows indicate neutrophils and arrowheads point to macrophages. Scale bar, 40 μm. (b) MPO activity was measured in wounds treated with CCN1-WT, CCN1-D125A mutant or PBS as above to evaluate neutrophil content (n=4 for treatment). (c) Expression ofIl-1βwas analysed by qRT–PCR (n=4 per treatment) and normalized to cyclophilin E. (d) Excisional wounds inLeprdb/dbmice were treated with PBS or recombinant CCN1 protein (0.2 mg ml−1, 50 μl per dose) daily from day 5 to day 8 and wound tissues harvested on day 9. (N=9 per treatment). Representative images of wound sections stained with H&E or anti-Ly6G showed efficient clearance of neutrophils in CCN1-treated wounds but not in PBS-treated controls. Scale bar, 100 μm. (e) MPO activity was measured in wounds ofLeprdb/dbmice after CCN1 treatment, indicating significant decrease in neutrophils (n=6 per treatment). (f)Ccn1mRNA levels in wounds ofLeprdb/dbmice was analysed by qRT–PCR (n=4 per time point). Statistical analyses were conducted using one-sided two-samplet-tests; NS, not significant (P>0.05). Protein lysates from these wounds were analysed by immunoblotting (g). Data expressed as mean±s.d. in triplicate determinations. Figure 8: CCN1 accelerates neutrophil clearance in slow-healing wounds. ( a ) Wounds of Ccn1 D125A/D125A mice were treated with recombinant WT CCN1 protein (0.2 mg ml −1 , 50 μl per dose) or PBS at day 6 and wound tissues were harvested at day 7, sectioned and stained with H&E. ( n =4 per treatment). Representative images were shown. Arrows indicate neutrophils and arrowheads point to macrophages. Scale bar, 40 μm. ( b ) MPO activity was measured in wounds treated with CCN1-WT, CCN1-D125A mutant or PBS as above to evaluate neutrophil content ( n =4 for treatment). ( c ) Expression of Il-1β was analysed by qRT–PCR ( n =4 per treatment) and normalized to cyclophilin E. ( d ) Excisional wounds in Lepr db/db mice were treated with PBS or recombinant CCN1 protein (0.2 mg ml −1 , 50 μl per dose) daily from day 5 to day 8 and wound tissues harvested on day 9. ( N =9 per treatment). Representative images of wound sections stained with H&E or anti-Ly6G showed efficient clearance of neutrophils in CCN1-treated wounds but not in PBS-treated controls. Scale bar, 100 μm. ( e ) MPO activity was measured in wounds of Lepr db/db mice after CCN1 treatment, indicating significant decrease in neutrophils ( n =6 per treatment). ( f ) Ccn1 mRNA levels in wounds of Lepr db/db mice was analysed by qRT–PCR ( n =4 per time point). Statistical analyses were conducted using one-sided two-sample t -tests; NS, not significant ( P >0.05). Protein lysates from these wounds were analysed by immunoblotting ( g ). Data expressed as mean±s.d. in triplicate determinations. Full size image Chronic non-healing or slow-healing wounds, including diabetic wounds, are often associated with prolonged or exacerbated inflammation, and excessive neutrophils have been reported in chronic pressure and venous ulcers [7] , [9] , [45] . Delayed wound healing with prolonged inflammation and neutrophil persistence is also reported in wounds of Lepr db/db mice, which carry an inactivating mutation in the leptin receptor gene and develop obesity and diabetes [8] . To investigate the activity of CCN1 in a diabetic context, excisional wounds of Lepr db/db mice were treated with daily administration of CCN1 protein from days 5 to 8 and analysed on day 9 ( Fig. 8d,e ). H&E staining showed inflammatory cell accumulation in PBS-treated control wounds, but not in CCN1-treated wounds ( Fig. 8d ). Immunostaining for Ly6G confirmed that the robust neutrophil accumulation was eliminated by CCN1 treatment in Lepr db/db wounds ( Fig. 8d ). Correspondingly, CCN1 treatment results in a dramatic reduction (>5-fold) in MPO activity in Lepr db/db wounds to the level similar to that of unwounded skin ( Fig. 8e ). Next, we assessed whether defects in neutrophil clearance in Lepr db/db wounds might be related to impaired Ccn1 expression. In contrast to significant increases in Ccn1 mRNA and protein in WT wounds ( Fig. 1a,b ), Ccn1 mRNA in Lepr db/db wounds showed only marginal increases on wounding that did not reach statistical significance ( Fig. 8f ). Moreover, the total CCN1 protein actually decreased on wounding in Lepr db/db mice, possibly due to a protease-rich environment in which neutrophils are aberrantly accumulated ( Fig. 8g ). Thus, there is a deficiency in Ccn1 expression in Lepr db/db wounds, leading to the accumulation of neutrophils. These results underscore the importance of CCN1 in promoting neutrophil efferocytosis in wound healing, suggesting a therapeutic potential for CCN1 in the treatment certain types of slow-healing wounds including diabetic wounds. Restoration of tissue integrity and homeostasis following injury to the skin is of vital importance, as the integument provides the first barrier against invading microbes and pathogens. Acute inflammation occurring immediately after injury plays a critical role for host defense and debridement of necrotic tissues, although deregulated inflammation or its persistence can cause further tissue damage and lead to chronic non-healing wounds. Impaired wound healing causes considerable morbidity in afflicted patients, and is a leading cause of diabetes-related amputations [46] . Thus, effective management of inflammation resolution is critical to wound care, and targeting excessive neutrophil activity has been proposed for treating chronic wounds such as venous ulcers [45] . Here we have uncovered a critical role for CCN1 in triggering efferocytosis of neutrophils by macrophages to promote the resolution of inflammation in skin wounds. CCN1 appears to be the first bridging molecule identified to play this role in cutaneous wound healing. Moreover, application of CCN1 accelerates neutrophil clearance in diabetic mouse wounds, suggesting a therapeutic potential for CCN1 in the treatment of certain types of impaired wound healing. To dissect the functions of CCN1 through distinct integrins, we have constructed an allelic series of knockin mice in which Ccn1 is replaced by alleles expressing CCN1 mutants unable to bind specific integrins. This approach circumvents the embryonic lethality of Ccn1 -null mice due to cardiovascular defects [34] , and avoids potential limitations in cell type-specific deletions as CCN1 may be secreted by diverse cell types in the tissue microenvironment. In skin wound healing, analysis of Ccn1 DM/DM knockin mice expressing CCN1 unable to bind α 6 β 1 /α M β 2 led to the discovery that CCN1 controls fibrosis through triggering myofibroblast senescence by engagement of α 6 β 1 (ref. 28 ), and studies on Ccn1 D125A/D125A mice reported herein revealed a critical function in promoting the resolution of inflammation through efferocytosis. Interestingly, fibroblast-specific deletion of Ccn1 , even in combination with deletion of the homologous family member Ccn2 , did not result in any change in wound closure rate [47] , suggesting that CCN1 produced from various cell types in the wound microenvironment adequately compensates for the loss of fibroblast-derived CCN1. Indeed, CCN1 is expressed in macrophages [48] , neutrophils ( Supplementary Fig. S2 ), endothelial cells [33] and fibroblasts [28] . No apparent defect in macrophage function was noted in Ccn1 DM/DM knockin mice, even though CCN1 can induce gene expression in macrophages through α M β 2 in culture [49] , suggesting that inflammatory cytokines or regulators other than CCN1 may prevail in regulating macrophage gene expression in the cutaneous wound. Multiple efferocytosis receptors and bridging molecules have been described, and they may play differential roles in various developmental and pathological contexts depending on their cell type specificity and time course of expression. For example, both Gas6 and Protein S contribute to the phagocytosis of photoreceptor outer segments by retinal pigment epithelial cells, but no other efferocytosis defect was observed among a myriad of phenotypes in Gas6, Protein S and TAM receptor mutant mice [25] , [50] . Mice lacking TSP-1, a bridging molecule, exhibit impaired angiogenesis in cutaneous wound healing but efferocytosis defect has not been reported [51] . Likewise, MFG-E8-null mice show reduced angiogenesis in skin wound healing without notable efferocytosis defect [52] . Indeed, whereas MFG-E8 is critical for the elimination of apoptotic B cells in the germinal centres [53] and mammary epithelial cells during mammary gland involution [54] , MFG-E8 is downregulated in virtually all inflammatory conditions and inflammation-related pathologies [55] , suggesting that it may not participate in neutrophil elimination. CCN1 binds to α v β 3 /α v β 5 on macrophages, PS on apoptotic neutrophils and α 6 β 1 on myofibroblasts through its vWC, TSR and CT domains, respectively, to exert distinct functions during wound healing ( Fig. 9 ). Since CCN family proteins emerged through evolution by exon shuffling [26] , [27] , it appears likely that this process recombined various structural domains from extracellular matrix proteins to confer unique functions governing multiple aspects of wound healing. CCN1 is known to dampen and resolve fibrosis in the maturation phase of wound healing by inducing myofibroblast senescence [28] . Our current findings suggest the possibility that CCN1 might further contribute to the restriction of fibrosis by promoting efferocytosis of apoptotic myofibroblasts. In support of this hypothesis, we found that CCN1 can promote macrophage engulfment of apoptotic fibroblastic cells ( Supplementary Fig. S10c ), and apoptotic myofibroblasts have been associated with restriction of fibrosis [56] . 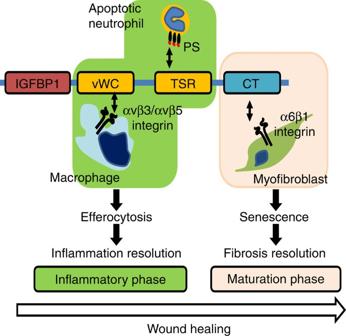Figure 9: A proposed schematic model for CCN1 actions in cutaneous wound healing. CCN1 serves distinct functions at different phases in wound healing through distinct structural domains. In the inflammatory phase, CCN1 acts as a bridging molecule to stimulate neutrophil clearance by binding integrins αvβ3/αvβ5in macrophages through its vWC domain and PS in apoptotic cells through its TSR domain. In the maturation phase, CCN1 functions to dampen and restrict fibrosis by triggering myofibroblast senescence by binding integrin α6β1through its CT domain28. Figure 9: A proposed schematic model for CCN1 actions in cutaneous wound healing. CCN1 serves distinct functions at different phases in wound healing through distinct structural domains. In the inflammatory phase, CCN1 acts as a bridging molecule to stimulate neutrophil clearance by binding integrins α v β 3 /α v β 5 in macrophages through its vWC domain and PS in apoptotic cells through its TSR domain. In the maturation phase, CCN1 functions to dampen and restrict fibrosis by triggering myofibroblast senescence by binding integrin α 6 β 1 through its CT domain [28] . Full size image Since CCN1 can induce angiogenesis through interaction with integrin α v β 3 in endothelial cells [35] , [36] , it is not surprising that Ccn1 D125A/D125A mice also exhibited impaired angiogenesis during wound healing. These knockin mice show reduced CD31-positive endothelial cells, fewer vessel-associated pericytes and diminished expression of angiogenesis-related genes ( Supplementary Fig. S6 ). However, neutrophil depletion rectified many of the wound-healing defects by accelerating wound closure, improving angiogenesis and promoting granulation tissue formation ( Fig. 4 ), suggesting that neutrophil persistence, rather than impaired angiogenesis, underlies the wound healing defects in Ccn1 D125A/D125A mice. As there are multiple angiogenic factors in the wound microenvironment, it is possible that CCN1 plays a redundant or relatively minor role in regulating angiogenesis during wound healing, and the angiogenic defect in Ccn1 D125A/D125A mice may have been exacerbated by neutrophil persistence. However, since the angiogenesis and efferocytosis functions of CCN1 are mediated through the same integrin and cannot be separated by mutation, understanding the angiogenic role of CCN1 in wound healing may require further scrutiny. Diabetic wounds often suffer from enhanced inflammation and delayed healing, and Lepr db/db mice exhibit these phenotypes [8] , [40] . In contrast to WT mice in which Ccn1 expression is enhanced on wounding ( Fig. 1a,b ), Ccn1 mRNA is not significantly elevated in Lepr db/db wounds and CCN1 protein actually decreased on wounding ( Fig. 8f,g ), potentially due to robust protease activity produced by accumulated neutrophils [45] . Thus, Lepr db/db wounds appear to suffer from impaired Ccn1 expression, leading to a deficit in CCN1 function. Consistently, CCN1 therapy of cutaneous wounds in Lepr db/db mice efficiently eliminated excess accumulation of neutrophils ( Fig. 8 ). Since these results are obtained in Lepr db/db mice, the specific role of CCN1 in normal and impaired human wounds remains to be determined. It is interesting to note that the CCN1-D125A mutant protein can inhibit efferocytosis in a dominant-negative manner ( Fig. 5d ), most likely by sequestering neutrophils through PS binding but being unable to bridge them to macrophages. Thus, cleavage of CCN1 through its protease-sensitive central hinge region between domains II and III [57] in certain pathological contexts may potentially generate CCN1 fragments that inhibit efferocytosis in a dominant-negative manner ( Fig. 7e ). For example, CCN1 is cleaved in lung epithelial cells from patients with COPD [58] , a disease in which impaired efferocytosis has been observed [15] . Whether CCN1 plays a critical role in efferocytosis in other inflammatory or pathological contexts beyond cutaneous wound repair is currently unknown. In this regard, it is noteworthy that aberrant Ccn1 expression has been reported in myriad inflammatory conditions, including sepsis [59] , inflammatory bowel disease [60] , [61] , rheumatoid arthritis [62] , COPD [63] , cholestasis [64] and cardiac injury repair [65] . It will be important to assess whether the opsonin function of CCN1 is important in these contexts. Moreover, CCN1 controls fibrosis by inducing senescence not only in skin wounds, but also in liver injuries induced by either hepatotoxin or cholestasis [29] , indicating that the role of CCN1 in tissue injury repair is potentially wide-ranging and not limited to cutaneous wounds. Prolonged inflammation is the hallmark of non-healing wounds, including diabetic wounds, pressure ulcers and venous ulcers [1] , [66] . Excessive neutrophils contribute to impaired healing, and thus wound closure in diabetic mice was accelerated by 50% on neutrophil depletion [40] . Here we show that CCN1 treatment leads to effective neutrophils removal in slow-healing wounds, including wounds of Ccn1 D125A/D125A and in Lepr db/db diabetic mice ( Fig. 8 ). These findings suggest a potential therapeutic value in the application of CCN1 in certain types of non-healing wounds [45] . Since CCN1 plays multiple and disparate roles in wound healing ( Fig. 9 ), the possibility that application of CCN1 in wound care may both accelerate inflammation resolution and dampen fibrosis and reduce scarring clearly warrants further investigation. CCN1 proteins and reagents Recombinant CCN1 and mutant proteins (D125A, DM, CCN1-I.II, CCN1-ΔCT and D125A-ΔCT) were produced using a baculovirus expression system in insect cells and purified by ion-exchange or immunoaffinity chromatography [30] , [32] . Rabbit polyclonal antibodies against CCN1 were raised against the CCN1 vWC domain [67] . Rabbit and mouse IgGs, echstatin and lipopolysacharide were from Sigma. RGDSP and RGESP peptides were from Bachem. Function-blocking mAbs against mouse integrin β 1 (KM16), α v (RMV-7), β 3 (2C9-G3), α v β 3 (23-C6) and β 5 (KN52) were from eBioscience. Recombinant murine interleukin-4 were from R&D Systems. Horse radish peroxidase (HRP)-conjugated anti-mouse and anti-rabbit secondary antibodies were from Amersham Biosciences. Biotin-conjugated goat anti-rabbit IgG, biotin-conjugated goat anti-rat IgG antibody and streptavidin-conjugated HRP were from Invitrogen. Animals and analysis of cutaneous wound healing Animal protocols were approved by the Institutional Animal Care and Use Committee of the University of Illinois at Chicago. Two independent lines of Ccn1 D125A/D125A mice (A5 and F5) were generated in a svJ129-C57BL/6 mixed background ( Fig. 2a ) and backcrossed more than six times into the C57BL/6 background; results from both lines were similar. Genetically diabetic mice (BKS.Cg-m+/+ Lepr db /J) were from Jackson Laboratories, and intercrossed to yield homozygous db/db mice. Typically, 10–12-week-old male mice with similar body weight ( ∼ 25–28 g for C57BL/6 mice) were used for cutaneous wound healing. Mice were anaesthetized with i.p. injection of ketamine/xylazine (100 mgkg −1 i.p.) and the dorsum of each mouse was clipped free of hair. Full-thickness excisional wounds through panniculus carnosus were created with a 6-mm biopsy punch (Miltex) and left open during the healing process [28] . For healing kinetic studies, digital images of wounds were taken and wound diameters were measured using Photoshop CS2 (Adobe). For histological analyses, wound tissues were snap-frozen in optimum cutting temperature compound (Tissue-Tek) and sectioned serially (7-μm thickness) using a Leica CM1950 UV cryostat. Alternatively, wound tissues were embedded in paraffin and sections were stained with H&E or probed with anti-Ly6G rat mAb (BD Pharmingen; 1A8, 1:100 dilution) or anti-CD68 rabbit polyclonal antibody (Abcam, 1:100 dilution), followed by biotin-conjugated goat anti-rat IgG secondary antibody coupled with streptavidin-HRP with 3,3′-Diaminobenzidine (Sigma) as substrate, and counterstained with haematoxylin. Apoptosis in wounds was detected using anti-activated caspase-3 polyclonal antibody (Cell Signaling) and visualized under fluorescence microscopy (Leica DM4000B). For western blot analysis, wound tissues were homogenized in radioimmunoprecipitation assay (RIPA) buffer (50 mM Tris-Cl pH 7.2, 150 mM NaCl, 0.1% SDS, 0.5% Na-deoxycholate, 1% Triton-X-100 and protease inhibitors cocktail) using polytron homogenizer, followed by sonication. Cellular senescence was evaluated by senescence-associated β-galactosidase staining of wound tissues [28] . Antisense oligonucleotide treatment Antisense oligonucleotide (AS-ODN) against Ccn1 was prepared in PBS and injected intradermally (200 μg per wound) into full-thickness excisional wounds on indicated days. Sense oligonucleotides (sense-ODN) were used as control. The sequences of oligonucleotides are: antisense, 5′- GCAGGCACGGGGCAGGTGG -3′ and sense, 5′- CCACCTGCCCGCTGCCTGC -3′. MPO assay The samples from freshly isolated wound tissues were prepared as described [68] , and MPO assay was performed in assay buffer (50 mM hexadecyl trimethyl ammonium bromide, 0.167 mg ml −1 of O-dianisidine dihydrochloride and 0.0005% hydrogen peroxide). MPO activity (absorbance) was measured using plate reader (Lab System, Multiscan MS) at 450 nm. Purified human MPO (Sigma) was used to generate a standard curve. Data were expressed as absorbance per wound weight. RNA isolation and qRT–PCR Skin wounds or cultured bone marrow-derived macrophages were homogenized using TRIzol reagent (Invitrogen) and total RNA was isolated using RNeasy Mini Kit (Quiagen). Total RNA (2 μg) was reverse transcribed to cDNA using MMLV-Reverse Transcriptase (Promega), and quantitative reverse transcription-PCR (qRT–PCR) was performed with the iCycler Thermal Cycler (Bio-Rad) using iQ SYBR Green Supermix (Bio-Rad). The specificity of qRT–PCR was confirmed by agarose gel electrophoresis and melting-curve analysis. A housekeeping gene ( cyclophilin E ) was used as an internal standard. The primers used are listed in Supplementary Table 1 . Isolation of bone marrow-derived macrophages and neutrophils Murine neutrophils and macrophages were isolated from bone marrow of either WT or Ccn1 D125A/D125A mice as described with modifications [69] , [70] . For neutrophil isolation, the resuspended bone marrow in Hank’s balanced salt solution (5 ml) was carefully layered over 62% Percoll (5 ml, Amersham) and centrifuged at 1,000 g for 30 min. After the gradient centrifugation, a cloudy layer containing neutrophils was removed from on top of the Percoll layer and resuspended in RPMI media for culture. An aliquot of cell suspension ( ∼ 20 μl) was spread on to the slide glass to assess the purity of isolated neutrophils by Giemsa staining (Sigma). For macrophages, the bone marrow cells were resuspended in macrophage complete media (DMEM/F12 with 20% (v/v) L-929 cells conditioned media), counted, and 4 × 10 5 cells were plated in sterile plastic petri dish (100 mm) and incubated in 37 °C in 5% CO 2 for 7 days with medium being refreshed on day 3 for full differentiation into macrophages. The macrophages differentiation was checked using F4/80 immunostaining. Efferocytosis assay Bone marrow-derived macrophages (10 5 cells per well) from either WT or Ccn1 D125A/D125A mice were plated on 12-well culture dish 1 day before the assay and labelled with CellTracker Green 5-chloromethylfluorescein diacetate (CMFDA; 5 μM, Invitrogen). Neutrophils were aged for 16 h and then incubated at 55 °C for 2 h before use as substrate for efferocytosis. Aged neutrophils (5 × 10 5 cells per well) were labelled with DAPI (10 mg ml −1 ) and incubated with macrophages for 60 or 90 min. Where indicated, CCN1 was preincubated with neutrophils for 1 h before incubation with macrophages. After incubation, cells were washed with ice-cold PBS four times fixed with 4% paraformaldehyde for 5 min. Efferocytosis was measured using the fluorescence microscopy by counting macrophages containing >2 neutrophils in 12 randomly selected high-powered fields and efferocytosis index was expressed as a percentage positive macrophages over total counted ( ∼ 300 cells). For inhibition of efferocytosis, PS-containing liposomes were prepared as described [22] and preloaded on to CCN1 for 30 min. For fibroblasts efferocytosis, human normal skin fibroblasts (1077SK; ATCC CRL-2094) were cultured, labelled with CellTracker Blue 4-chloromethyl-6,8-difluoro-7-hydroxycoumarin (5 μM, Invitrogen) and induced to undergo apoptosis by exposure to staurosporine (1 μM; Invitrogen) for 16 h. Efferocytosis assay was performed as described above. Depletion of neutrophils in mice Neutrophils depletion was achieved as described [38] . In brief, anti-Ly6G mAb (hybridoma clone# RB6-8C5; originally developed by Dr Robert I. Coffman, DNAX Research Institute, Palo Alto, CA and obtained from Dr David Sibley, Washington University, St Louis, MO) was produced under serum-free conditions using a CELLine bioreactor (CL350; Argos technologies, IL). Anti-Ly6G mAb (0.5 mg per mouse) was delivered in a single i.p. injection 1 day before wounding. Neutrophils depletion was confirmed by whole blood count on day 2 post wounding. Immunofluorescence Frozen wound tissues were cold acetone-fixed, washed in PBS-Tween-20 (PBST) and incubated in normal goat serum blocking solution containing 2% goat serum, 1% bovine serum albumin, 0.1% cold fish skin gelatin, 0.1% Triton-X-100, 0.05% Tween-20, 0.05% sodium azide and 0.01M PBS (pH 7.2) for 1 h. For labelling, the single primary antibody or antibody mixes were applied for 16 h at 4 °C. After washing (5 × ) in PBST, slides were incubated with the secondary antibodies (Texas Red-conjugated anti-rabbit IgG and Alexafluor488-conjugated anti-rat IgG; Invitrogen, 1:500 dilution each) for 30 min, followed by washing (5 × ) in PBST. DAPI was used as counterstain (1 mg ml −1 ). Fluorescence images were acquired using a Leica DM4000B microscope and processed with Photoshop CS2 (Adobe). Primary antibodies used for immunofluorescence staining are followed: anti-Ly6G rat mAb (1A8; BD Pharmingen, 1:100 dilution), anti-CD68 rat mAb (FA-11; Abcam, 1:100 dilution), anti-CD68 rabbit polyclonal antibody (Abcam, 1:200 dilution), anti-CD31 rat mAb (MEC 7.46; Abcam, 1:200 dilution), anti-NG2 rabbit polyclonal antibody (AB5320; Millipore, 1:100 dilution), anti-desmin rabbit polyclonal antibody (Abcam, 1:200 dilution), anti-CK14 mouse mAb (LL002; Abcam, 1:200 dilution), anti-vimentin rabbit polyclonal antibody (Abcam, 1:200 dilution) and anti-CCN1 rabbit polyclonal antibody (from the house, 1:200 dilution). Cell migration assay Human immortalized HaCaT keratinocytes were plated on to non-TC-treated dishes that were precoated with rat tail collagen I (4.3 mg ml −1 ; BD Bioscience) and serum starved for 48 h. Cells were pretreated with mitomycin C (10 μg ml −1 ; Sigma) for 30 min, followed by treatment of human epidermal growth factor (10 ng ml −1 ) or recombinant CCN1 protein (either WT or D125A mutants; 2 μg ml −1 each). Cell migration was assessed after 48 h and quantified using Image J software. PS binding Standard binding assays usually coat plastic wells with phospholipids, followed by the addition of binding protein and immunodetection of the binding protein. However, CCN1 is a cell adhesion molecule and characteristically coats plastic surfaces efficiently even in a short incubation period, making it impossible to detect specific binding using this protocol. Thus, we precoated 96-well plates with serial dilution of CCN1 proteins (WT, DM and D125A) and laminin at 4 °C overnight. After washing with PBST (2 × ), uncoated area was blocked with bovine serum albumin (10 mg ml −1 ) for 1 h. A total of 300 ng of PS was then added to each well for 1 h, followed by washing with PBST (3 × ). Anti-PS mAb (Abcam; 1 μg per well) was added, and standard enzyme-linked immunosorbent assay protocol was employed using 3,3′,5,5′-Tetramethylbenzine as a substrate and measured at OD 450 nm (ref. 20 ). Alternatively, lipid membranes (Echelon biosciences) were incubated overnight with CCN1 proteins (WT, CCN1-N, CCN1-ΔCT and D125A-ΔCT; 10 μg each), and anti-CCN1 vWC antibodies were used for detection. Co-immunoprecipitation Murine macrophages (Raw264.7) were treated with recombinant WT CCN1 protein or CCN1-D125A (5 μg each) for 30 or 60 min. Cells were lysed with RIPA buffer at 4 °C for 4 h with gentle agitation, followed by centrifugation at 13,000 g for 30 min. Supernatants were carefully removed and incubated with 1 μg of either anti-CrkII (C-18; Santa Cruz), anti-p130 Cas (C-20; Santa Cruz), or anti-FAK (C-20; Santa Cruz) at 4 °C for overnight. Protein G agarose beads (5 μl; Amersham) were added for 1 h, then followed by centrifugation at 10,000 g for 1 min. Pellets were washed four times with RIPA buffer and lysates were prepared with Laemmli sample buffer (3 × ). Western blot analyses of immune complex were performed for anti-CrkII (C-18; 1:1,000 dilution), anti-p130 Cas (C-20; 1:1,000 dilution), anti-FAK (C-20; 1:500 dilution) and anti-phophoFAK (Tyr397; #3283, Cell Signaling; 1:250 dilution). Images have been cropped for presentation. Full-size images are presented in Supplementary Fig. S11 . GTP-Rac1 pull-down assay Activated, GTP-bound Rac1 was detected using Rac1 activation assay kit (Cell Biolabs Inc.) according to the manufacturer’s instruction. In brief, bone marrow-derived macrophages were treated with CCN1-WT or CCN1-D125A (4 μg each) for 60 min. Cells were then washed with cold PBS twice and lysed. The cell lysates were incubated with 20 μg of PAK1-PBD (p21-binding domain of p21-activated protein kinase) agarose for 1 h at 4 °C. The precipitation of GTP-Rac1 was detected by immunoblotting. Statistics Results are expressed as the mean±s.d., and statistical analysis was performed by one-sided two-sample t -tests and one-way analysis of variance (for multiple group comparison) with Bonferroni post hoc tests. A P <0.05 was considered significant. All experiments were performed in triplicate, unless otherwise indicated. How to cite this article: Jun, J.-I. et al . The matricellular protein CCN1 mediates neutrophil efferocytosis in cutaneous wound healing. Nat. Commun. 6:7386 doi: 10.1038/ncomms8386 (2015).